Mesoporous bismuth ferrite with amplified magnetoelectric coupling and electric field-induced ferrimagnetism Coupled ferromagnetic and ferroelectric materials, known as multiferroics, are an important class of materials that allow magnetism to be manipulated through the application of electric fields. Bismuth ferrite, BiFeO 3 , is the most-studied intrinsic magnetoelectric multiferroic because it maintains both ferroelectric and magnetic ordering to well above room temperature. Here we report the use of epitaxy-free wet chemical methods to create strained nanoporous BiFeO 3 . We find that the strained material shows large changes in saturation magnetization on application of an electric field, changing from 0.04 to 0.84 μ b per Fe. For comparison, non-porous films produced using analogous methods change from just 0.002 to 0.01 μ b per Fe on application of the same electric field. The results indicate that nanoscale architecture can complement strain-layer epitaxy as a tool to strain engineer magnetoelectric materials. Multiferroic materials have been the focus of much research due to their potential application in spintronic- and memory-based devices [1] , [2] . These materials, which combine ferromagnetism and ferroelectricity, allow the control of one parameter through the other [3] . Few materials couple both properties in a single phase and even fewer achieve this at room temperature. Bismuth ferrite, BiFeO 3 (BFO), is one of the few examples of a room temperature multiferroic, and for this reason it has been widely researched [4] , [5] , [6] , [7] , [8] , [9] , [10] , [11] , [12] , [13] , [14] , [15] , [16] , despite the fact that it is mostly antiferromagnetic with <2° spin canting and thus a low saturation magnetization ( M S ) [4] , [5] . A few hexaferrites, including Sr 3 Co 2 Fe 24 O 41 , also show room temperature multiferroic properties [17] , [18] , but this work focuses on the better-understood BFO system with a goal of learning how nanoscale architecture, and particularly the flexibility of nanoscale networks, can be used to control magnetoelectric coupling. We build on recent experiments that used a variety of methods to tune the properties of BFO. For example, epitaxy has been used to amplify magnetic polarizations in BFO and other materials by the introduction of lattice strains [5] , [19] , [20] , [21] , [22] , [23] . Epitaxial strain has also been used to convert materials that are neither ferroelectric nor ferromagnetic to multiferroics at low temperatures [24] . For BFO in specific, thin films engineered with epitaxial strain show M S values up to 0.5 Bohr magnetons ( μ b ) per Fe (refs 22 , 25 ), which is substantially higher than the bulk value of 0.05 μ b per Fe (refs 22 , 26 ). High values of 0.2–0.3 μ b per Fe were also observed in highly strained mixed-phase (rhombohedral:super-tetragonal) epitaxial BFO [23] . While epitaxial strain in BFO has provided a fruitful method to tune materials properties, bulk, thin film, and nanostructured BFO have been made using a number of methods [12] , [14] , [19] , [27] , [28] , [29] , [30] , [31] , [32] , [33] , [34] , [35] , [36] , [37] . 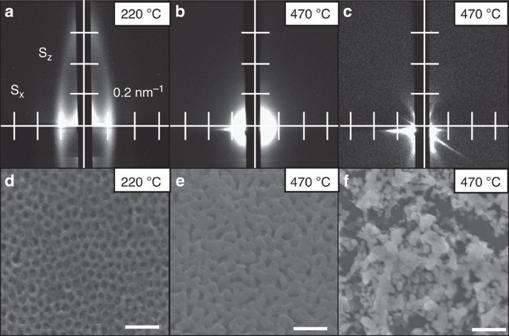Figure 1: Scanning electron microscopy and 2D-SAXS measurements of BFO mesoporous films. Frameworks are: amorphous (a,d), crystallized with partial retention of ordered porosity (b,e) and crystallized with loss of ordered porosity (c,f). All scale bars are 100 nm. SAXS patterns were collected at an angle of incidenceβ=0.1°. Supplementary Table 1 summarizes a portion of this previous work, comparing M s values for BFO synthesized in different ways. Of particular note is the work on sol-gel-derived BFO that also showed high M s values. In this case, however, the high values were attributed not to strain engineering in the material, but to the presence of Fe in the 2 + oxidation state and accompanying oxygen vacancies [14] . Here we present an alternative approach for producing thin-film BFO with anisotropic strain states using templated porous nanostructures that show both comparatively high magnetization and, more importantly, large changes in magnetization on application of an electric field. Our porous BFO films were produced by the co-assembly of ampiphilic diblock co-polymer templates with sol-gel type inorganic precursors; thermal processing was used to decompose the polymer and crystallize the BFO, leaving a crystalline film with a homogeneous, nanoporous architecture (see Methods section for synthetic details) [38] . As control samples, non-templated sol-gel (dense) films were also prepared for comparison with the porous films. Dense samples were prepared using the same inorganic precursor solution used for the porous film; however, the polymer template was not added in the dense film case. The dense and porous films were then annealed at the exact same temperatures and using the same heating rates to insure comparable crystallization of the films. Previous studies of mesoporous thin films composed of magnetostrictive cobalt ferrite revealed that flexing and contracting of the pores on high-temperature crystallization produced anisotropic strain states that resulted in magnetic anisotropy [39] . In this report, we demonstrate that strains achieved in templated nanoporous BFO films allow for magnetoelectric coupling that exceeds that reported previously for epitaxial thin-film counterparts in samples that do not contain significant levels of oxygen vacancies. Structural characterization Scanning electron microscopy studies of porous but amorphous BFO frameworks indicate that the materials have homogeneous porosity throughout the film ( Fig. 1b ). Two-dimensional small-angle X-ray scattering (2D-SAXS) further indicates that amorphous films have scattering maxima consistent with a disordered cubic pore network. Both in-plane and out-of-plane q values are consistent with previous reports employing related polymer templates ( Fig. 1a ) [39] . The elliptical nature of the diffraction pattern indicates that the pores are anisotropic, with significant out-of-plane pore shrinkage during heating [39] that is not balanced by in-plane contraction because the films are anchored to the silicon substrate. On further thermal annealing to achieve crystallization of the framework, some rearrangement of the mesoporous structure is observed ( Fig. 1d ), but the porosity remains homogeneous. This partial disordering results in a loss of out-of-plane scattering in 2D-SAXS measurements because of the finite film thickness, but in-plane scattering is still present ( Fig. 1c ). If templated films are heated too long during crystallization, nanoscale homogeneity and SAXS scattering are lost, and cracks form in the film to release in-plane strain ( Fig. 1e,f ). Similar cracks form if the films are too thick, even with optimal heating, because strain energy within the film becomes greater than the interfacial adhesion ( Supplementary Fig. 1 ). Figure 1: Scanning electron microscopy and 2D-SAXS measurements of BFO mesoporous films. Frameworks are: amorphous ( a , d ), crystallized with partial retention of ordered porosity ( b , e ) and crystallized with loss of ordered porosity ( c , f ). All scale bars are 100 nm. SAXS patterns were collected at an angle of incidence β =0.1°. Full size image For all BFO films, phase-pure Perovskite-structured materials were achieved, as confirmed by high-angle X-ray diffraction (XRD) measurements. 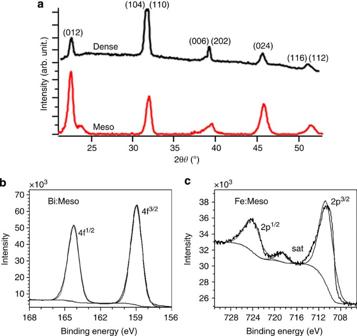Figure 2: Powder XRD and XPS measurements of BFO mesoporous and dense films. (a) Powder XRD obtained on mesoporous (bottom curve, red) and dense (top curve, black) BFO thin films. Peaks correspond phase-pure BFO (JCPDS #01-071-2494). (b,c) XPS core level spectra of mesoporous BFO films. Bi 4f (b) and Fe 2p (c) peaks are shown for both samples. All data can be fit to the 3+ oxidation state of both Bi and Fe. Nearly identical data were obtained for dense (non-porous) BFO films (seeSupplementary Fig. 3for details). Figure 2a shows the diffraction patterns for both the dense and nanoporous samples; no peaks from contaminating phases were observed. The polycrystalline films also possess no preferred domain orientation, as determined by 2D-XRD ( Supplementary Fig. 2 ). To further confirm the phase purity of the BFO films, X-ray photoelectron spectroscopy (XPS) data were collected on both porous ( Fig. 2b,c ) and dense ( Supplementary Fig. 3 ) films. For both samples, the data can be fit to a single 3+ oxidation state for both the Fe and the Bi. In specific, the Fe peak is centred at 710.8 eV, in good agreement with the expected value of 711 eV for Fe 3+ , suggesting phase purity and a low-enough level of oxygen vacancies that they were not detected via XPS [40] . These data thus provide good evidence that the high M s values reported below do not arise from oxygen vacancies, as seen in some other sol-gel-derived materials, but more likely stem from strain effects, in closer analogy to epitaxial BFO systems [22] , [23] , [25] . Figure 2: Powder XRD and XPS measurements of BFO mesoporous and dense films. ( a ) Powder XRD obtained on mesoporous (bottom curve, red) and dense (top curve, black) BFO thin films. Peaks correspond phase-pure BFO (JCPDS #01-071-2494). ( b , c ) XPS core level spectra of mesoporous BFO films. Bi 4f ( b ) and Fe 2p ( c ) peaks are shown for both samples. All data can be fit to the 3+ oxidation state of both Bi and Fe. Nearly identical data were obtained for dense (non-porous) BFO films (see Supplementary Fig. 3 for details). Full size image Magnetoelectric coupling Piezo-force microscopy (PFM) measurements allow us to visualize the ferroelectric properties of these nanoporous films, using the PFM tip as one electrode and a conducting substrate as the other. Concentric boxes of alternating polarization were written into the porous BFO films, illustrating the presence of switchable ferroelectric dipole moments that are stable at room temperature ( Fig. 3a ). The piezo-force curve in Fig. 3b shows that the application of a modest bias can be used to switch the ferroelectric domain. Magnetic properties of mesoporous and non-templated sol-gel (dense) BFO films were investigated via SQuID magnetometry. Magnetization curves ( M versus H ) for both mesoporous and dense BFO films revealed M S values of 0.04 and 0.001 μ b per Fe, respectively ( Supplementary Fig. 4 ); the higher value for the porous samples likely result from unpaired surface spins [7] . All systems were ferrimagnetic at room temperature with small spin canting angles, as noted by small but measurable values for both the coercive widths and the saturation magnetization. 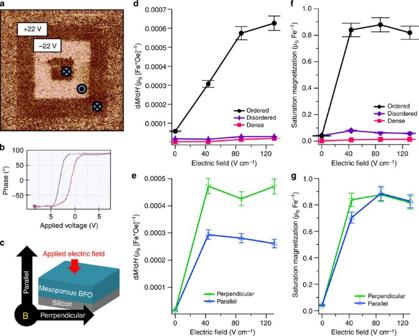Figure 3: Magnetoelectic characterization of mesoporous and dense BFO films. (a) PFM phase image showing response to positive and negative fields for mesoporous BFO. (b) Phase versus applied voltage curve for the BFO sample froma. (c) Schematic of the electric and magnetic field orientations used ford–g. Magnetic measurements displaying the effects of an electric field on dM/dH(d,e) and the saturation magnetization (f,g) for ordered mesoporous, dense and disordered mesoporous structures (d,f) and for mesoporous films oriented parallel and perpendicular to the external magnetic field (e,g). Error bars calculated from the uncertainty in sample volume. Figure 3: Magnetoelectic characterization of mesoporous and dense BFO films. ( a ) PFM phase image showing response to positive and negative fields for mesoporous BFO. ( b ) Phase versus applied voltage curve for the BFO sample from a . ( c ) Schematic of the electric and magnetic field orientations used for d – g . Magnetic measurements displaying the effects of an electric field on d M /d H ( d , e ) and the saturation magnetization ( f , g ) for ordered mesoporous, dense and disordered mesoporous structures ( d , f ) and for mesoporous films oriented parallel and perpendicular to the external magnetic field ( e , g ). Error bars calculated from the uncertainty in sample volume. Full size image Theoretical calculations on unstrained BFO predict an increase in magnetic susceptibility (d M /d H ) in BFO perpendicular to an applied electric field direction and a decrease in susceptibility parallel to it, because electric poling establishes a magnetic easy axis orthogonal to the electric polling direction [19] , [41] . We measured d M /d H by poling the films in a modest electric field, followed by measurement of the magnetic properties ex situ in a SQuID magnetometer. On poling, d M /d H , measured perpendicular to the poling direction in ordered mesoporous BFO increased 10-fold, from 5.8 × 10 −5 μ b *(Fe·Oe) −1 to 6.3 × 10 −4 μ b *(Fe·Oe) −1 ( Fig. 3d ). With the same applied field, the change in the dense sample was minimal. In contrast to theoretical predictions, however, an increase in d M /d H was also observed for porous films measured with the magnetic field applied parallel to the electric field poling direction ( Fig. 3e ), though the increase is smaller than that observed in the perpendicular direction. One would expect an increase in susceptibility for magnetization perpendicular to the applied electric field and a decrease when the magnetic field is parallel to the applied electric field. This contradiction with theory can be explained by the observation that a large part of the increase in the d M /d H values on electrical poling arises not from establishment of a magnetic easy axis oriented perpendicular to the applied electric field, but instead from an increase in the saturation magnetization ( M s ) on electric poling. Figure 3f,g shows the surprising result that application of modest external electric fields dramatically increased M S for the ordered mesoporous films, with values increasing from 0.04 to 0.84 μ b per Fe on application of just 44 V cm −1 . The change in M S is equivalent, measured either parallel or perpendicular to the applied field ( Fig. 3g ); this indicates that the increase arises from intrinsic changes in spin canting, rather than from the formation of a magnetic easy axis. In these nanoporous materials, we thus have two multiferroic coupling mechanisms active at once. The dominant mechanism is an increase in spin canting on application of an electric field. Superimposed on this isotropic increase in susceptibility are changes in MCA, which are standardly found in multiferroic BFO. The MCA changes favour a perpendicular relationship between the applied electric field and the magnetization direction. The result is that the magnetic susceptibility increases both parallel and perpendicular to the applied field, but to a larger extent in the perpendicular direction, as seen in Fig. 2e . The dense BFO shows much lower M S values, increasing from 0.002 to just 0.01 μ b per Fe on application of the same field. We also note that the low M s values in all unpoled samples preclude the possibility that iron oxide impurities or oxygen vacancies, as discussed above, from the sol-gel synthesis are the source of the high magnetization in poled samples. These M s values for electrically poled mesoporous BFO films demonstrate the highest values recorded for BFO films to date, greater even than values ranging from 0.2–0.5 μ b per Fe reported in epitaxially strained BFO thin films [23] , [25] . Indeed, this magnetization change corresponds to a magnetoelectric coupling constant α = μ 0 Δ M / E =1 × 10 −5 sm −1 , which is on par with composite systems and much larger than that expected for single phase materials [42] , [43] . While the numerical results are exciting, the role played by the nanoscale architecture in controlling this large magnetoelectric response is of more fundamental interest. When samples are crystallized with a loss of homogeneous nanoscale porosity and strain is released due to cracking ( Fig. 1e,f ), samples show little change in M s on electric poling, increasing only from 0.04 to 0.06 μ b per Fe ( Fig. 3f ). In addition, if significantly thicker films are made, the strain in the film will overcome the interfacial adhesion and the films will crack or delaminate from the substrate so that the strain is again released. This also results in a small change in M s for thicker films (see Supplementary Fig. 1 ), despite having a homogeneous, interconnected pore system. Anisotropic strain induced by flexible interconnected-nanoscale porosity, strongly bound to a rigid substrate thus appears to be key to the magnetoelectric coupling observed here. High-resolution XRD To probe the origin of the large magnetoelectric coupling in these BFO films, synchrotron-based high-resolution XRD studies were conducted. The bulk space group for BFO is R3c (ref. 44 ); however, for simplicity, planes are indexed in R3m, which is based on the cubic lattice. The (100), (110) and (1–10) lattices planes were investigated as a function of applied electric field to observe changes in the lattice. The latter pair of reflections provides a measure of the rhombohedral distortion from the cubic lattice. The cubic (110) splits from a single peak into the rhombohedral (110) (1–10) pair (JCPDS 01-071-2494). Since the samples are comprised of randomly oriented polycrystalline domains, all peaks could be observed in both in-plane and out-of-plane orientations, allowing us to use these peaks as a probe of the strain state of the porous BFO. The data in Fig. 4 show that the application of an external electric field induces permanent changes in the lattice spacings of mesoporous BFO, while dense BFO lattice spacings were essentially unaffected by electrical poling. The voltage range used for this experiment is similar to that used for SQuID studies ( Fig. 3 ), but slightly lower voltages were chosen to better overlap the region of maximum change in the magnetic susceptibility. For both porous and dense BFO samples, the three lattice planes were examined both perpendicular and parallel to the poling direction. Changes in all lattice planes are summarized in Supplementary Table 2 , and shifts in the (110) and (1–10) peaks displayed graphically in Fig. 4a,c for porous BFO and Fig. 4b,d for dense BFO. For the porous samples, all three lattice planes show an overall contraction on electrical poling. In contrast, the bulk samples show minimal change on application of an electric field; Supplementary Table 2 indicates ∼ 10 × greater change in d-spacing for mesoporous compared with dense samples. The large change for the mesoporous sample likely arises from increased flexibility of the porous framework. 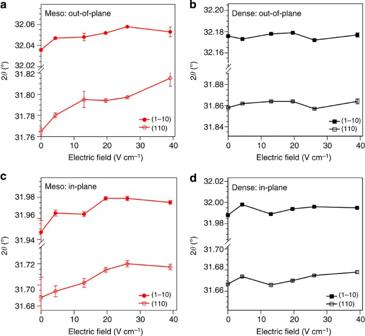Figure 4: High-angle synchrotron experiments of mesoporous and dense BFO films. The experiments display the shifts in peak position for out-of-plane (a,b) and in-plane (c,d) (110) and (1–10) lattice planes as a function of electric field. (All data reported assuming Cu K-α radiation). Error bars calculated as the s.d. of the reported peak position. Figure 4: High-angle synchrotron experiments of mesoporous and dense BFO films. The experiments display the shifts in peak position for out-of-plane ( a , b ) and in-plane ( c , d ) (110) and (1–10) lattice planes as a function of electric field. (All data reported assuming Cu K-α radiation). Error bars calculated as the s.d. of the reported peak position. Full size image In addition to the contraction, a reduction in splitting was observed for the out-of-plane (110) and (1–10) lattice planes for the porous samples ( Fig. 4a ). These planes, which are oriented parallel to the plane of the substrate, should most effectively couple to out-of-plane flexing of the nanoscale pores. The splitting in this peak arises from the rhombohedral distortion in BFO. Decreased splitting thus indicates that the rhombohedral angle, α , is tending back towards 90° for out-of-plane-oriented domains only, corresponding to a reduction of symmetry induced by the applied electric field. It is worth noting that the average in-plane and out-of-plane strains for the porous BFO are small, only ∼ 0.1–0.2% (tension) and ∼ 0.4–0.5% (compression), respectively. Lattice strains in epitaxial, lattice mismatched BFO and are reported as 1.4% (on SrTiO 3 ) and 4.8% (on LaAlO 3 ) in-plane tension [45] . Thus, the strains we are seeing in our porous films are much lower. This suggests that the enhanced magnetization observed here is due not just to the extent of lattice strain, but rather the nature of the strain. Indeed, theoretical calculations [20] have already concluded that no linear strain within a given symmetry unit cell can produce results like those seen here. This suggests that it is the symmetry lowering that is primarily responsible for the increase in M s in these films. To fully understand the results presented here, it is useful to summarize the trends across samples. Mesoporous samples before electrical poling show a slightly amplified magnetic moment compared with dense samples, which likely arise from unpaired surface spins [7] . For samples with more ordered pores, a large increase of this magnetic moment is observed on electric poling, apparently arising from field-induced anisotropic strains. Dense samples do not show either the initial amplification of magnetism or any significant increase on poling. Disordered porous samples and thick-film porous samples again have an initially elevated magnetization, as expected for a high surface area sample [7] but show no changes in magnetization on electrical poling. We thus hypothesize that because of the flexibility of porous materials, electric poling of the constrained interconnected pore system can effectively distort the lattice, reducing the rhombohedral symmetry. This results in increased spin canting and saturation magnetization in the ordered porous BFO. Thus, the combination of mechanically flexible pores bound to a rigid substrate, and an intrinsic multiferroic, where spin canting is directly coupled to structural distortions, are needed for the ferrimagnetic, multiferroic properties observed here. We showed above that porosity provides a powerful tool to strain engineer nanostructured materials. The high surface area of nanoporous materials also provides an opportunity to create intimately mixed composite materials as the pores can play host to a myriad of materials. As an example, mesoporous BFO films fabricated on platinized silicon wafers were electroplated with a ferromagnetic nickel phase. The electroplating technique successfully filled the pores and was non-destructive, as evidenced by TEM images ( Fig. 5 ) and energy dispersive spectroscopy to identify the phases. This proof-of-principal experiment lays the foundation for future work aimed at realizing intimately mixed composite materials [41] , [46] , [47] , [48] based on mesoporous frameworks. 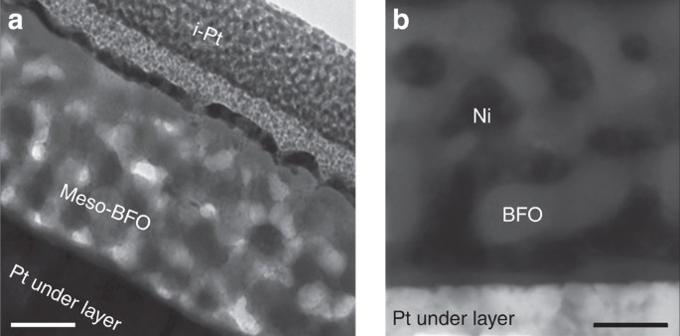Figure 5: Dark-field scanning transmission electron microscopy (STEM) images of nickel plated mesoporous BFO. Nickel can be electroplated into the porous framework, as determined by high-angle, annular dark-field STEM images. Both lower magnification—scale bar, 50 nm (a) and high-resolution images—scale bar, 20 nm (b) demonstrate complete pore filling. Phases were identified using energy dispersive spectroscopy. Figure 5: Dark-field scanning transmission electron microscopy (STEM) images of nickel plated mesoporous BFO. Nickel can be electroplated into the porous framework, as determined by high-angle, annular dark-field STEM images. Both lower magnification—scale bar, 50 nm ( a ) and high-resolution images—scale bar, 20 nm ( b ) demonstrate complete pore filling. Phases were identified using energy dispersive spectroscopy. Full size image Facile production of nanostructured BFO with electrically switchable, enhanced ferrimagnetism in thin-film format could be beneficial for a range of applications [1] , [2] , [3] . Porous materials thus offer interesting potential for strain engineering using wet chemical methods without the need for expensive epitaxy. Strain induced by porosity can be reproducibly generated and can be tuned, though not with the precision of epitaxial films [24] , by controlled thermal annealing [39] . The observation of electrically induced changes in both strain and M S in porous BFO further demonstrates novel magnetoelectric coupling not previously observed in epitaxially strained materials. This work thus adds to a growing body of results focused on using strain to convert antiferromagnetic BFO into a ferrimagnetic magnetoelectric material. At the same time, we open a new avenue for strain engineering using flexible nanoporous architectures. Materials and synthesis Bi(NO 3 ) 3 × 5H 2 O (99.9%) and Fe(NO 3 ) 3 × 9H 2 O (99.9%) were purchased from Sigma-Aldrich and used without further purification. H[(CH 2 CH 2 ) 0.67 (CH 2 (CH)CH 2 CH 3 ) 0.33 ] 89 -[OCH 2 CH 2 ] 79 OH (referred to as KLE-22) was used as the organic template. For a typical synthesis of mesoporous BFO, a scintillation vial was charged with Bi(NO 3 ) 3 × 5H 2 O (0.371 g), Fe(NO 3 ) 3 × 9H 2 O (0.310 g) and 2 ml anhydrous 2-methoxyethanol and allowed to stir for several hours. In a separate vial, the diblock co-polymer KLE-22 (0.085 g) was added to 1 ml ethanol and heated to 50 °C until completely dissolved. The two solutions were combined into a single vial and allowed to stir for further 2 h, filtered and were ready for deposition. Films were deposited via dip coating in a humidity-controlled environment (25–25%) at varying withdrawal rates (between 1 and 2 cm s −1 ) depending on the desired film thickness. Once deposited, the films are heated in air from 50 to 180 °C over a 3-h period, and are allowed to soak for 12 h. To achieve crystallization of the mesoporous films, further annealing is required; the films are heated in air to 475 °C at 4 °C min −1 , soaked for 1 min and removed immediately. Instrumentation and characterization In- and out-of-plane high-angle XRD, 2D-SAXS, FESEM (field emission scanning electron microscopy) and SQUID magnetometry were conducted to characterize the samples. Conventional high-angle XRD was measured using a D8-GADDS diffractometer from Bruker instruments (Cu-K α radiation). 2D-SAXS and angular-dependent high-angle XRD data were collected at the Stanford Synchrotron Radiation Laboratory using beam lines 1–4 and 7–2, respectively. FESEM images were obtained using a JEOL 6700F instrument. Magnetic measurements were carried out on a Quantum Design MPMS 5T SQUID magnetometer with RSO detection. Site-selective cross-sectional TEM sample preparation was performed using an Omniprobe lift-out on a dual-beam FEI Strata 400 focused ion beam. All high-resolution transmission electron microscopy and high-angle annular dark-field scanning transmission electron microscopy were performed on a JEOL 2100 operating at an accelerating voltage of 200 kV. PFM measurements were performed on a Dimension 5000 system operating in DC mode. XPS analysis was performed using a Kratos Axis Ultra DLD with a monochromatic (Al—Kα radiation) source. The charge neutralizer filament was used to control charging of the sample. A 20-eV pass energy was used with a 0.05-eV pass energy. Scans were calibrated using the C 1 s peak shifted to 284.8 eV. How to cite this article: Quickel, T. E. et al . Mesoporous bismuth ferrite with amplified magnetoelectric coupling and electric field-induced ferrimagnetism. Nat. Commun. 6:6562 doi: 10.1038/ncomms7562 (2015).